Catalytically active single-atom niobium in graphitic layers Carbides of groups IV through VI (Ti, V and Cr groups) have long been proposed as substitutes for noble metal-based electrocatalysts in polymer electrolyte fuel cells. However, their catalytic activity has been extremely limited because of the low density and stability of catalytically active sites. Here we report the excellent performance of a niobium–carbon structure for catalysing the cathodic oxygen reduction reaction. A large number of single niobium atoms and ultra small clusters trapped in graphitic layers are directly identified using state-of-the-art aberration-corrected scanning transmission electron microscopy. This structure not only enhances the overall conductivity for accelerating the exchange of ions and electrons, but it suppresses the chemical/thermal coarsening of the active particles. Experimental results coupled with theory calculations reveal that the single niobium atoms incorporated within the graphitic layers produce a redistribution of d -band electrons and become surprisingly active for O 2 adsorption and dissociation, and also exhibit high stability. Catalysts for the cathodic oxygen reduction reaction (ORR) are key components in polymer electrolyte fuel cells [1] . Noble metal-based catalysts have exhibited the most efficient catalytic performance; nevertheless, the high cost and scarcity, together with poor tolerance and instability, present two main challenges in the field: one is to improve the durability and efficiency of ORR catalysts; the other is the search for inexpensive and abundant alternative catalysts. Strategies for increasing the active sites, either by reducing the size of catalyst clusters [2] , [3] or by producing particles with high-index, externally exposed facets [4] , have been proven effective. Furthermore, single-atom catalysts of noble metals have shown better catalytic activities in comparison with those of subnanometre counterparts [5] , [6] , [7] , [8] , [9] . However, such noble metal catalysts, downsized to subnanometre or single-metal atoms, are structurally unstable. Even under inert conditions, their high reactivity would result in serious aggregation and coarsening, interfering with the density of active sites and limiting the catalytic durability and efficiency. Since Levy and Boudart [10] reported Pt-like features of tungsten carbide in several catalytic reactions, carbides of groups IV through VI have become an important substitute for noble metal-based electrocatalysts because of their superior stability and low cost [10] , [11] . However, optimization of the catalyst size and/or surface structures to maximize the catalytic efficiency has limited their widespread adoption [12] . Moreover, there is a mystery surrounding the behaviour of subnanometre or even smaller clusters; it is unclear whether they will retain the catalytic characteristics or have better catalytic performance than their bulk counterparts. Herein we report a new class of carbide catalyst (denoted as Nb-in-C) synthesized by an arc-discharge approach ( Supplementary Fig. S1 ). Abundant single niobium atoms are found to be incorporated into onion-like carbon shells surrounding ~1.6 nm niobium carbide cores. To demonstrate the role of the single niobium atoms incorporated in the graphite layers in ORR, we also synthesize a structure consisting of similar niobium carbide particles (~2 nm ) encapsulated within graphite shells but with a much reduced number of incorporated single niobium atoms (denoted as NbC-in-C, see Supplementary Figs S2–S6 ) and compare its catalytic properties. Both structures are characterized at the atomic scale by microscopy and active sites corroborated by theoretical simulations. The results show that single niobium atoms incorporated in graphite layers are the sites of high catalytic activity responsible for the excellent ORR performance. Electrocatalytic performance for ORR The ORR properties were evaluated systematically in an Ag/AgCl three-electrode electrochemical cell. The Nb-in-C complex was deposited on a rotated-disk glassy carbon (GC) electrode (5.6 mm in diameter) to form a mass density of 60 μg cm −2 . The cyclic voltammetry curves of the Nb-in-C catalysts were recorded at room temperature and at a scan rate of 100 mV s −1 . As shown in Fig. 1a , O 2 reduction current exhibited a well-defined cathodic peak with onset potential of −0.13 V in O 2 -saturated 0.1 M KOH, whereas a featureless voltammetric current was observed within the potential range between −1.0 and +0.2 V in N 2 -saturated 0.1 M KOH. The featureless voltammogram is similar to that of amorphous/disordered carbon, which is ascribed to high-fraction carbon debris that was formed in the non-equilibrium evaporation–condensation process. Such debris has been confirmed by the low thermal oxidation temperature ( Supplementary Fig. S7 ) and Raman spectroscopy ( Supplementary Fig. S8 ). The electrocatalytic selectivity was further examined in O 2 -saturated 0.1 M KOH in the presence of methanol (3.0 M), showing no noticeable change in contrast to the case of O 2 -saturated 0.1 M KOH electrolyte. Such electrocatalytic activity and high selectivity of the Nb-in-C complex/GC electrode towards the ORR indicate a remarkably good ability to avoid crossover effects in polymer electrolyte fuel cells. 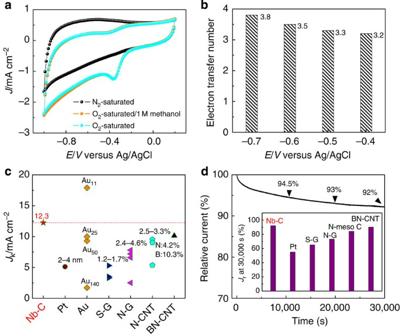Figure 1: Evaluation of ORR properties of Nb-in-C complex. (a) Cyclic voltammogram curves of ORR on Nb-in-C complex in a N2-saturated 0.1 M KOH solution, an O2-saturated 0.1 M KOH solution, with and without the addition of 1 M methanol (CH3OH), at a scan rate of 100 mV s−1. (b) The dependence of electron transfer number (n) on potential for the Nb-in-C complex. (c) Kinetic-limiting current density (Jk) at −0.5 V in comparison with that of currently reported studies. Note that theJkvalue of BN-CNT is calculated at −0.3 V and others are at −0.5 V. (d) Chronoamperometric response curve of the Nb-in-C complex recorded at 0.5 V in an O2-saturated 0.1 M KOH at a rotation rate of 1,600 r.p.m. The references of Pt, Au, S-G, N-G, N-CNT, BN-CNT and N-meso C represent commercial Pt nanoparticles14, Au clusters3, sulphur-doped graphene14, nitrogen-doped graphene14, nitrogen-doped19, nitrogen/boron-doped carbon nanotubes15and nitrogen-doped mesoporous carbon16, respectively. Figure 1: Evaluation of ORR properties of Nb-in-C complex. ( a ) Cyclic voltammogram curves of ORR on Nb-in-C complex in a N 2 -saturated 0.1 M KOH solution, an O 2 -saturated 0.1 M KOH solution, with and without the addition of 1 M methanol (CH 3 OH), at a scan rate of 100 mV s −1 . ( b ) The dependence of electron transfer number ( n ) on potential for the Nb-in-C complex. ( c ) Kinetic-limiting current density ( J k ) at −0.5 V in comparison with that of currently reported studies. Note that the J k value of BN-CNT is calculated at −0.3 V and others are at −0.5 V. ( d ) Chronoamperometric response curve of the Nb-in-C complex recorded at 0.5 V in an O 2 -saturated 0.1 M KOH at a rotation rate of 1,600 r.p.m. The references of Pt, Au, S-G, N-G, N-CNT, BN-CNT and N-meso C represent commercial Pt nanoparticles [14] , Au clusters [3] , sulphur-doped graphene [14] , nitrogen-doped graphene [14] , nitrogen-doped [19] , nitrogen/boron-doped carbon nanotubes [15] and nitrogen-doped mesoporous carbon [16] , respectively. Full size image To uncover the role of the Nb-in-C complex/GC electrodes during the ORR electrochemical process, polarization curves ( Supplementary Fig. S9a ) were measured at a scan rate of 5 mV s −1 and at various rotation rates ranging from 400 to 2,400 r.p.m. It is evident that the mass-transfer-limited current density was enhanced by an increase in the rotation rate, with an onset potential at approximately −0.13 V. Supplementary Fig. S9b shows the corresponding Koutecky–Levich (K–L) plots ( J −1 versus ω −1/2 ). The good linearity and parallelism of these plots indicate first-order reaction kinetics with respect to the concentration of dissolved O 2 . On the basis of the K–L plots, the electron transfer numbers ( n ) for ORR at different potentials were estimated to be 3.2~3.8 ( Fig. 1b ), which is comparable to other non-noble catalysts for the four-electron ORR; for examples, n =3.9 for N-doped carbon nanotubes (CNTs) ( [13] ), n =2.8~3.5 for N or S-doped graphene [14] , n =3.7 for B/N-doped CNTs ( [15] ) and n =3.89 for nitrogen-doped ordered mesoporous graphitic arrays [16] . The limiting current plateau at around −0.5~−0.7 V is not as obvious as seen for Pt-based catalysts. This phenomenon has been reported in many carbon-based catalysts [15] , [16] , [17] , [18] . It is recognized that the nanoporous microstructure of catalysts provides three-dimensional continuous channels for O 2 penetration due to the capillary force and applied potential. The slower ORR dynamics of non-noble metal catalysts compared with Pt-based catalysts result in excess residual O 2 reduction at high overpotentials. The slight incline at high overpotentials is thus ascribed to the porous structure of the Nb-in-C complex. As shown in Fig. 1c , the kinetic-limiting current density ( J k ) was calculated to be 12.3 mA cm −2 at −0.5 V, higher than that of commercially Pt-C/GC [14] , graphene [14] , CNTs ( [15] , [19] ) and ultra small Au clusters (except Au 11 ) [3] . The chronoamperometric curves recorded at −0.40 V and a rotation rate of 1,600 r.p.m. in an O 2 -saturated 0.1 M KOH solution have been used to evaluate the durability of the Nb-in-C complex. The measurements after 30,000 s indicated that the residual current still remained at 92%, which is comparable to that of other currently reported catalysts [14] , [15] , [19] ( Fig. 1d ). Atomic-scale microstructure characterization To understand the catalytic activity and stability of the Nb-in-C complex, the structure was initially characterized using a scanning electron microscope operated at a voltage of 30 kV (Hitachi S-4700). As shown in Supplementary Fig. S4a , the sample presented an aggregated yet porous structure. To reveal the atomic-scale microstructure, we employed a fifth-order aberration-corrected scanning transmission electron microscope (STEM, Nion-UltraSTEM100), coupled with an electron energy-loss spectrometer (EELS; Gatan Enfina spectrometer). The low accelerating voltage of 60 kV ensured a non-destructive characterization and, in particular, was critical to avoid the electron beam-induced sintering of subnanometre clusters and single atoms [20] . From the representative bright-field image in Fig. 2a , it is clearly observed that the carbon matrix was mainly composed of onion-like graphite structures and highly defective, layered graphitic material. Using powder X-ray diffraction analysis ( Fig. 2b ), the components of Nb-in-C complex were further verified to be graphitic carbon and niobium carbide, with significant lattice expansion, which appears important for improving catalytic properties [11] . The total fraction of the carbon component confirmed by thermogravimetric analysis (TGA) was estimated to be ~86.3 wt% ( Supplementary Fig. S7a ). 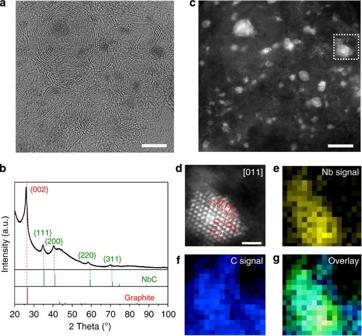Figure 2: Microstructural characterizations of Nb-in-C complex. (a) High-magnification bright-field image showing nanosized onion-like carbon shells. Scale bar, 5 nm. (b) X-ray diffraction scan of Nb-in-C powder. (c) ADF image of the same region asFig. 2a, exhibiting subnanometre niobium carbide particles (bright features) that are invisible in the bright-field image. Scale bar, 5 nm. (d) Enlarged ADF image of a representative niobium carbide particle marked inFig. 2c(scale bar, 1 nm.) and (e–g) its EELS mapping of Nb and C components. Figure 2: Microstructural characterizations of Nb-in-C complex. ( a ) High-magnification bright-field image showing nanosized onion-like carbon shells. Scale bar, 5 nm. ( b ) X-ray diffraction scan of Nb-in-C powder. ( c ) ADF image of the same region as Fig. 2a , exhibiting subnanometre niobium carbide particles (bright features) that are invisible in the bright-field image. Scale bar, 5 nm. ( d ) Enlarged ADF image of a representative niobium carbide particle marked in Fig. 2c (scale bar, 1 nm.) and ( e–g ) its EELS mapping of Nb and C components. Full size image The annular dark-field (ADF) images reflect the mass-thickness contrast in which the regions with higher-density and/or heavier elements generate brighter contrast [20] , [21] . Thus, the niobium clusters and atoms in the ADF mode exhibit brighter contrast as compared with the carbon matrix. In the same region of Fig. 2a , a corresponding ADF image ( Fig. 2c ) further reveals a more heterogeneous dispersion of subnanometre niobium carbide clusters and single niobium atoms than can be seen in the bright-field image. Furthermore, a niobium carbide cluster encapsulated with carbon shells were directly identified by the EELS analysis and the composition visualization, as seen in Fig. 2d–g and Supplementary Fig. S10 . 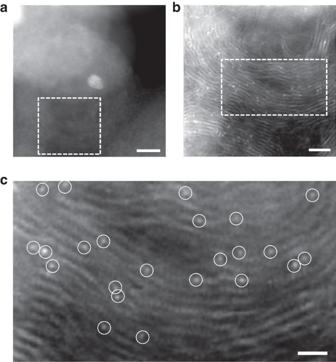Figure 3: Direct observation of single niobium atoms in a Nb-in-C nanocapsule. (a) ADF image of a single Nb-in-C nanocapsule, in which one can see that a ~2.5 nm niobium carbide cluster was encapsulated by an onion-like carbon shell. Scale bar, 5 nm. (b) Enlarged image of the region marked inFig. 3a, revealing a high density of graphitic defects in the carbon shell. Scale bar, 2 nm. It is noteworthy that there are many single niobium atoms (bright dots) doped in the carbon shell, which is further magnified inFig. 3c, as highlighted by white circles. Scale bar, 1 nm. Figure 3a shows an ~2.5nm niobium carbide cluster encapsulated in a hollow onion-like carbon shell. The graphitic shell with distorted {002} planes contains pronounced ripples and mesoporous defects, which were most likely derived from the rapid cooling process [13] . The high-magnification image in Fig. 3b shows single niobium atoms uniformly dispersed in the graphitic shells. The stability of these single niobium atoms under electron beam irradiation ( Supplementary Movie 1 ), compared with that of niobium atoms on the surface of a niobium carbide cluster ( Supplementary Movie 2 ), indicates that they are trapped in the graphitic layers rather than on the outer surface of graphite shells. Figure 3c shows that the single niobium atoms (marked by the white circles) occupy substitutional sites of the carbon atom planes rather than intercalation sites between carbon planes. Quantum mechanical calculations indicate that the most energetically favourable site for single niobium atoms is a trivacancy site in the carbon layer, in which the niobium atom sits 0.035 nm higher than the carbon plane ( Supplementary Figs S11 and S12 ). The consistency between the experimental observations and theoretical predictions strengthens our hypothesis that the single niobium atoms are located within the graphitic skeleton. Figure 3: Direct observation of single niobium atoms in a Nb-in-C nanocapsule. ( a ) ADF image of a single Nb-in-C nanocapsule, in which one can see that a ~2.5 nm niobium carbide cluster was encapsulated by an onion-like carbon shell. Scale bar, 5 nm. ( b ) Enlarged image of the region marked in Fig. 3a , revealing a high density of graphitic defects in the carbon shell. Scale bar, 2 nm. It is noteworthy that there are many single niobium atoms (bright dots) doped in the carbon shell, which is further magnified in Fig. 3c , as highlighted by white circles. Scale bar, 1 nm. Full size image The graphitic shells of the Nb-in-C complex was analysed by TGA and Raman spectroscopy. The onset oxidation temperature occurred at 314 °C ( Supplementary Fig. S7a ), which was significantly lower than that of other carbon allotropes, such as 1~3 layer graphene (~450 °C) ( [22] ), C 60 (~500 °C) ( [23] ), multi-walled CNTs (MWCNTs; ~700 °C) ( [23] ), boron-doped MWCNTs (~770 °C) ( [24] ), nitrogen-doped MWCNTs (~450 °C) ( [25] ) and bulk graphite crystals (846 o C) ( [26] ). The lower oxidation temperature reflects the defective nature of this form of carbon, partly induced by niobium incorporation, which provides active sites for O 2 absorption. The existence of such defective sites is also suggested by the high I D /I G ratio (0.98) seen in the Raman spectrum ( Supplementary Fig. S8 ). Origin of the electrocatalytic activity Several important studies on niobium carbonitride with partial oxidation, associated with Nb 2 O 5 species on the surface, have suggested that the surface oxide is the origin of catalysis [27] , [28] . However, the atomic-scale characterization indicates that there is no surface oxide on the samples and, thus, the origin of catalysis in our materials is the niobium–carbon complexes rather than the oxide. In particular, there is no evidence of any O edge at 532 eV in the EELS spectroscopy, indicating the particles are not oxidized (see Supplementary Fig. S10 and the Discussion). To distinguish the catalytic roles of single niobium atoms and niobium carbide clusters, we tested the NbC-in-C sample containing encapsulated niobium carbide particles but with an order-of-magnitude reduced number of incorporated single niobium atoms. The NbC-in-C sample was obtained under a moderate cooling condition, as discussed in detail in the Supplementary Information . The statistical diameter of ~1,000 clusters in the NbC-in-C is ~2 nm, only slightly larger than the ~1.6 nm diameter seen in Nb-in-C. Supplementary Fig. S5a,b,c shows the magnified STEM images of the niobium carbide clusters in NbC-in-C, indicating that all the observed niobium carbide clusters are encapsulated in the graphitic layers. Supplementary Fig. S5d,e,f shows there are almost no single niobium atoms found incorporated in the graphitic layers. These images indicate that the single niobium atoms are rarely trapped in the graphitic layers when moderate cooling rates are used. Electrocatalytic characterization of NbC-in-C was carried out to reveal its ORR characteristics, as shown in Supplementary Figs S13 and S14 . On the basis of the K–L plots, the number of electrons transferred per O 2 molecule ( n ) for ORR is 1.65~2.44 at the recorded potentials, indicating that the ORR process for NbC-in-C is dominated by a 2e − reduction pathway. The kinetic-limiting current density ( J k ) value for NbC-in-C is 0.912 mA cm −2 at −0.5 V, an order of magnitude lower than that for Nb-in-C ( J k =12.3 mA cm −2 ). Thus, it is deduced that the superior 4e − ORR catalytic characteristics of Nb-in-C are mainly due to the presence and stability of the large number of single niobium atoms. The origin of the catalytic characteristics of carbides of groups IV through VI is ascribed to the redistribution of d -band electrons of the metal atoms. This reconstruction is calculated to result in an increased density of states (DOS) near the Fermi surface [11] . As the niobium carbides in the Nb-in-C complex ranged from ~2 nm down to single niobium atoms, we investigated the catalytic activity as a function of particle size. The niobium carbide clusters were modelled as niobium carbide octahedra with eight niobium-terminated {111} facets combined with a single niobium atom incorporated in a carbon trivacancy site. DFT calculations provide isosurfaces of the charge densities of three configurations in a small energy window near the Fermi surface ( Fig. 4a ). These plots show that the d -electrons located both at external corners and edges of low-coordinated niobium atoms in the carbide particles, as well as the electrons on the single niobium atoms incorporated into the graphitic layers, result in an increased DOS near the Fermi surface. This was further quantitatively demonstrated by analysis of the DOS at the Fermi level at niobium atoms in various configurations as shown in Fig. 4b , presenting much higher values for ultra small clusters and single niobium atoms compared with a niobium-terminated {111} surface and bulk niobium. 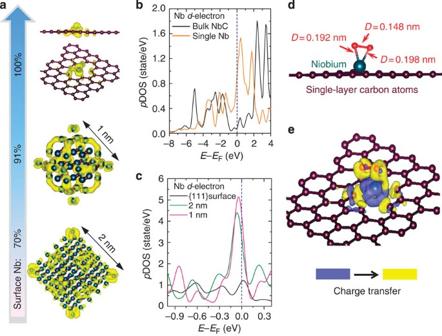Figure 4: Theoretical simulations of the catalytic origins. (a) Isosurface of the charge-density distribution in the energy windowEF−0.01 eV toEFof the niobium carbide clusters with edge sizes of 2 and 1 nm, and the single niobium atom doped in a carbon layer. (b,c) Thed-electron DOS for the niobium atoms at the corner of clusters, as well as the doped single niobium atom. The DOS of perfect Nb-terminated NbC{111} and bulk niobium carbide are listed for comparison. The DOS are normalized by the total number of Nb atoms. (d) Geometrical arrangement of adsorbed O2on the single niobium site. (e) Isosurface of the difference in electron density before and after O2adsorption. Charge flows from the niobium atom (blue) into the O atoms (yellow). Figure 4: Theoretical simulations of the catalytic origins. ( a ) Isosurface of the charge-density distribution in the energy window E F −0.01 eV to E F of the niobium carbide clusters with edge sizes of 2 and 1 nm, and the single niobium atom doped in a carbon layer. ( b , c ) The d -electron DOS for the niobium atoms at the corner of clusters, as well as the doped single niobium atom. The DOS of perfect Nb-terminated NbC{111} and bulk niobium carbide are listed for comparison. The DOS are normalized by the total number of Nb atoms. ( d ) Geometrical arrangement of adsorbed O 2 on the single niobium site. ( e ) Isosurface of the difference in electron density before and after O 2 adsorption. Charge flows from the niobium atom (blue) into the O atoms (yellow). Full size image To reveal the catalytic ability of these single niobium atoms in ORR, a simplified model consisting of an O 2 molecule adsorbed on the surface of the single niobium atom-doped graphite layer was characterized using spin-polarized first-principles calculations. Unlike the normal adsorption at precious metal surfaces, the O 2 molecule prefers side-on adsorption ( Fig. 4d ). The diatomic adsorption effectively weakens the O–O bonding. The O–O bond length and stretching frequency are computed to be 0.148 nm and 513 cm −1 , significantly weaker than that of O 2 at a perfect Pt {111} surface (0.143 nm and 690 cm −1 ) ( [29] ), which thus facilitates the O–O dissociation. Furthermore, the calculated adsorption energy of atomic oxygen is 0.80 eV for the Nb in a graphene trivacancy configuration, which is comparable to 0.71–0.83 eV for Pt n clusters ( n =2~6 atoms), which implies that the single-atom niobium–carbon complex should exhibit noble metal-like performance for the ORR ( [30] ). From the isoenergy surfaces of electron densities differences shown in Fig. 4e , an obvious charge transfer from the niobium atom to the two O atoms can be observed, associated with a filling of π * anti-bonding states. This is the origin of the relatively low O–O dissociation energy barrier. These atomic-scale insights confirm that the low-coordinated and single niobium atoms are the most active catalyst sites. Experimental studies have unambiguously confirmed that O 2 can penetrate into the graphitic layers and react at specific doping sites; for example, the graphite-based materials doped by light atoms [13] , [14] , [15] , [16] , [19] , [31] , [32] , [33] , [34] . The catalytic characteristics of the doped carbon are found to be dramatically enhanced compared with undoped carbon. Our observations indicate that niobium-doped graphite, with its high density of defects, also allows easy O 2 penetration and reaction at single niobium sites. Smaller particles usually have reduced chemical and structural stability, which results from unavoidable particle coarsening during the catalytic reaction process. However, the niobium carbide clusters and single niobium atoms in our materials are encased in onion-like carbon shells that not only enhance the overall conductivity for accelerating the exchange of ions and electrons during the ORR process, but also suppress the chemical/thermal coarsening of the particles. This structure effectively ensures the electrochemical stability of catalytically active single-atom sites. In addition, the large number of graphitic defects improves O 2 permittivity and possibly has a role as catalytically active sites for O 2 reduction [13] , [14] , [15] , [16] , [19] , [31] , [32] , [33] . These combined advantages make the Nb-in-C complex particularly suitable for practical electrochemical ORR catalysis. Obviously, such niobium–carbon structures also have the potential to be used in other catalysis reactions such as the decomposition of ammonia [35] , the catalytic CO oxidation reactions [36] and the catalytic oxidation of sulphides [37] . Our modified arc-discharge equipment can be continuously operated by circulating the methane gas to reach a productivity of 50–100 g per hour, which is attractive for practical industrial applications. We therefore believe that our results would be of major interest to a wide range of catalysis applications. This study presents a new approach for stabilizing metallic single atoms and subnanometre clusters, and thus opens up the possibility for developing highly efficient and durable electrocatalysts based on other transition metal carbides. Sample synthesis The schematic diagram of the modified arc-discharge equipment is shown in Supplementary Fig. S1 . A high-purity niobium rod forms the anode, attached to a water-cooled copper stage for rapid sample cooling, whereas the upper carbon rod serves as the cathode. The chamber is first evacuated to reach ~10 −2 Pa and, subsequently, methane (CH 4 ) is introduced as a gaseous carbon source to reach 0.1 × 10 5 Pa. Evaporating the niobium rod by arc-discharge at ~30 V and ~90 A conditions results in a simultaneous decomposition of methane. The current and voltage are controlled by adjusting the distance between the niobium rod and the carbon rod for continuous stable operation. During this evaporation process, we have noticed that the carbon rod has negligible loss compared with the carbon decomposed from the methane. The arc-evaporated niobium and decomposed carbon form black smoke and simultaneously deposit on the cool walls of the chamber. The as-fabricated product is collected after about ~6 h. Characterization The microstructures of Nb-in-C and NbC-in-C complexes were analysed using a Hitachi S-4700 transmission/scanning electron microscopy operated at a voltage of 30 kV. STEM imaging and EELS were performed using an aberration-corrected STEM (Nion-UltraSTEM100) operating at a low accelerating voltage of 60 kV. The achievable spatial resolution using this fifth-order aberration-corrected microscope at 60 kV is ~1.2 Å. ADF images were obtained using 58–200 mrad detector half-angle. EEL spectra were collected using a Gatan Enfina spectrometer with a collection half-angle of 48 mrad. The energy resolution of the EELS spectrum measured from the zero-loss full width at half-maximum was 0.3 eV. A Siemens D-500 X-ray diffractometer with CuK α ( λ =0.154 nm) radiation at a voltage of 30 kV and a current of 30 mA was used to study the phase structure of the products at a scan step of 0.2°. The oxidation behaviours were investigated by TGA in an air atmosphere at a heating rate of 10 o C min −1 from 50 to 900 o C. Electrochemical test Electrochemical measurements were conducted using a three-compartment electrochemical cell. A saturated Ag/AgCl electrode and a Pt plate were used as reference and counter electrodes, respectively. The Nb-in-C complex was deposited on a GC rotating disk electrode (RDE) (5.6 mm in diameter, mirror polished) and dried under vacuum at room temperature. Nafion water solution (10 μl, 0.1 wt%) was deposited and evaporated to form a protective film. The cyclic voltammetry curves of catalysts were recorded at room temperature and at a scan rate of 100 mV s −1 . Three kinds of electrolytes were used in this study, that is, N 2 -saturated 0.1 M KOH, O 2 -saturated 0.1 M KOH and O 2 -saturated 0.1 M KOH in the presence of methanol (3.0 M).By measuring the RDE current-potential curves at various rotating speeds, the limited diffusion currents ( J K ) and electron transfer number ( n ) were calculated based on the K–L equations: where J is the measured current density, J K and J L are the kinetic- and diffusion-limiting current densities, ω is the angular velocity of RDE, n is the overall number of electrons transferred in oxygen reduction, F is the Faraday constant ( F =96,485 C mol −1 ), C 0 is the bulk concentration of O 2 , ( C 0 =1.2 × 10 −3 mol cm −3 ), ν is the kinematic viscosity of the electrolyte ( ν =0.01 cm 2 s −1 ), and D 0 is the diffusion coefficient of O 2 in 0.1 M KOH (1.9 × 10 −5 cm 2 s −1 ). Theoretical simulation The calculations have been performed using the Vienna ab initio simulation pack [38] . The projected augmented wave method and the Perdew–Wang generalized gradient approximation were used to describe electron–ion interactions. A thermal broadening of 0.1 eV was applied to improve the convergence of the self-consistent procedure and non-spin polarization was employed for all calculations, except the O 2 adsorption simulation with plane-wave cut-off energy of 50 Ry. For bulk NbC with NaCl-type structure, a 20 × 20 × 20 Monkhorst–Pack grid was used for the integration of the elemental unit cell over the Brillouin zones. The calculated equilibrium lattice constant for NbC was 4.46 Å, which agrees well with the experiment value (4.40 Å). The niobium-terminated surface is calculated to be the energy-favourable perfect NbC (111) surface. The NbC clusters with different sizes were located in the 25 Å × 25 Å × 25 Å simulation box, and the stable configurations were obtained through full relaxation according to the Hellmann–Feynman forces. To investigate the energy-favourable local atomic configuration of a single niobium atom on the graphitic layers, the atomic configurations ( Supplementary Figs S11–S12 ) were fully relaxed and the formation energy was calculated, where E Nb+C , E Nb and E c-layer are the potential energies of a niobium-doped graphene layer (or three atomic-layer graphite), a free niobium atom and a defective graphene layer (or three atomic-layer graphite), respectively.We considered all the possible configurations of a single Nb atom at a single vacancy, bivacancy, trivacancy or quad vacancy of carbon atomic layer. In all the configurations that we proposed, shown in Supplementary Figs S11 and S12 , the configuration (Nb+G@V 3 ) shown in Fig. 4d is the most probable site for O 2 catalytic reduction. Accordingly, we studied the catalytic activity of an O 2 molecule absorbed on this most probable configuration (Nb+G@V 3 ) of a single niobium atom–carbon layer. The free O 2 molecule was added close to the niobium–carbon layer without any artificial assumption, such as the adsorption sites. By optimizing both the structure and energy at 300 K, the O 2 molecule seeks its most favourable absorption site and configuration, and bonds with the Nb atom after only ~100 ps (20,000 steps) simulation. The bond length of the O 2 molecule was calculated to be 1.22 Å and the atomic configuration of O 2 adsorbed on the single niobium site was calculated, including spin polarization. How to cite this article: Zhang, X. et al . Catalytically active single-atom niobium in graphitic layers. Nat. Commun. 4:1924 doi: 10.1038/ncomms2929 (2013).